CSN-mediated deneddylation differentially modulates Ci155proteolysis to promote Hedgehog signalling responses The Hedgehog (Hh) morphogen directs distinct cell responses according to its distinct signalling levels. Hh signalling stabilizes transcription factor cubitus interruptus (Ci) by prohibiting SCF Slimb -dependent ubiquitylation and proteolysis of Ci. How graded Hh signalling confers differential SCF Slimb -mediated Ci proteolysis in responding cells remains unclear. Here, we show that in COP9 signalosome ( CSN ) mutants, in which deneddylation of SCF Slimb is inactivated, Ci is destabilized in low-to-intermediate Hh signalling cells. As a consequence, expression of the low-threshold Hh target gene dpp is disrupted, highlighting the critical role of CSN deneddylation on low-to-intermediate Hh signalling response. The status of Ci phosphorylation and the level of E1 ubiquitin-activating enzyme are tightly coupled to this CSN regulation. We propose that the affinity of substrate–E3 interaction, ligase activity and E1 activity are three major determinants for substrate ubiquitylation and thereby substrate degradation in vivo . In developing tissues, morphogens are produced and secreted from different sources to build concentration gradients that serve as positional information, directing cells of different distances away from the source to adapt distinct fates [1] , [2] . To pattern complex tissues with precision, it is conceivable that the intracellular signalling level should scale to the morphogen gradient [3] , [4] , [5] , [6] . The Hedgehog (Hh) family proteins are evolutionarily conserved. As secreted morphogens, they have been implicated in patterning the formation of vertebrate face, spinal cord and digits, and Drosophila eyes, wings and several others [4] , [7] , [8] , [9] , [10] . In Drosophila developing wing discs, Hh signalling involves at least three distinct mechanisms in regulating the zinc-finger transcription factor cubitus interruptus (Ci), namely, blocking the proteolysis of the transcriptional activator full-length Ci (Ci 155 ) (refs 11 , 12 , 13 ), enhancing Ci 155 nuclear partitioning [14] , [15] , [16] , [17] and transactivation activity [18] , [19] , [20] . In the absence of Hh signalling, Ci 155 is partially proteolysed to generate the transcriptional repressor Ci (Ci 75 ). Ci 155 proteolysis requires consecutive phosphorylation of Ci 155 by protein kinase A (PKA) [21] , [22] , glycogen synthase kinase 3β (GSK3β) [23] , [24] and casein kinase I (CKI) [23] , [25] , resulting in a high affinity for the F-box protein Slimb of the SCF Slimb ubiquitin (Ub) ligase complex for ubiquitylation [13] , [26] , [27] . Although it had been demonstrated that Hh signalling stabilizes Ci 155 by precluding phosphorylation-dependent ubiquitylation of Ci 155 (refs 23 , 24 ), how graded Hh signals are translated into graded Ci 155 proteolysis is not clear. The Ub E3 ligase activities of SCF (skp1-cullin- F -box protein) and other types of cullin–RING ligases (CRLs) are regulated by the conjugation of the Ub-like polypeptide Nedd8 onto the cullin scaffold component of CRLs, a process known as neddylation [28] , [29] . Genetic analyses performed in neddylation pathway mutants of various species indicate that Nedd8 modification of cullins is essential for CRL activities [27] , [30] , [31] , [32] , [33] , [34] . For example, neddylation is required for SCF Slimb -mediated Ci 155 proteolysis in cells not receiving Hh, thus suppressing Hh-mediated gene activation [12] . Nedd8 conjugation at a conserved carboxy-terminal lysine in all cullin proteins facilitates the binding of the RING domain-containing protein Rbx1/ROC1 that recruits Ub-loaded E2s [29] , [35] . Furthermore, neddylation induces a conformational change of the Cul5 carboxy terminus, which facilitates the transfer of Ub onto substrates [36] . Consistently, neddylation reduces the K m for E2 binding to CRL and increases the K cat for substrate ubiquitylation, thus increasing the processivity of ubiquitylation [37] . It has been estimated that neddylation of SCF allows the processive addition of more than four Ubs in a productive substrate–SCF encounter [38] . The Nedd8 moiety on cullins can be deconjugated by the COP9 signalosome (CSN) complex, thus inactivating CRL ligase activities [39] , [40] . Similar to other reversible protein modifications, neddylation and deneddylation of cullins occur dynamically in vivo [30] , [41] . Little is known whether dynamic deneddylation of CRLs is indeed critical to the substrate stability through modulating the extent of substrate ubiquitylation in vivo . To better understand the role of deneddylation in Ci 155 stability, in response to the Hh gradient, in this study, we used the Drosophila wing disc as a model in which cells display distinct responses to the Hh morphogen because of their positions. We analysed the SCF Slimb -mediated Ci 155 proteolysis in mutants for CSN , GSK3β ( sgg in Drosophila ), Cul1 , slimb and E1 Ub-activating enzyme uba1 . Taken together, our results suggest that deneddylation by regulating SCF Slimb activity protects a portion of partially phosphorylated Ci 155 from proteolysis, thus establishing the low-threshold Hh signalling responses. CSN deneddylation regulates the protein stability of Slimb Whereas neddylation of cullins promotes CRL activities, deneddylation of cullins also promotes substrate degradation, mainly through protecting cullins and substrate receptors from neddylation-induced degradation [42] , [43] , [44] , [45] , [46] . To test whether protection of substrate receptors by deneddylation is a general rule, we first examined the protein stability of Slimb, a substrate receptor for the SCF complex that ubiquitylates several substrates including Ci 155 (refs 13 , 47 ). Mutant clones for the CSN catalytic subunit CSN5 ( CSN5 null ) were generated in third-instar wing discs that also carry the myc-slimb transgene under the control of the ubiquitous tubulin promoter. In CSN5 null cells, the protein level of Myc-Slimb is diminished (arrow in Fig. 1a ), suggesting that the CSN is required to stabilize Slimb in vivo . In contrast, neddylation promotes Myc-Slimb turnover, as Myc-Slimb accumulates to high levels in cells homozygous for Nedd8 AN015 (arrow in Fig. 1b ). To test whether the SCF-Slimb interaction is essential for neddylation-mediated Slimb turnover, we examined the protein stability of Myc-SlimbΔfbx that cannot be incorporated into the SCF complex because of the truncation of the F-box [47] . In contrast to the full-length Slimb, the protein levels of SlimbΔfbx in CSN5 null mutant and neighbouring wild-type cells are indistinguishable ( Fig. 1c ). Taken together, we conclude that the substrate receptor Slimb, when incorporated into the SCF complex, is regulated by neddylation-induced degradation. However, neddylation-induced degradation of substrate receptors is unlikely a general rule, as the protein level of the Flag-conjugated F-box protein Archipelago (Flag-Ago) is unaltered in CSN5 null cells ( Fig. 1d ), suggesting that neddylation and deneddylation regulate the protein stability of some but not all of the SCF substrate receptors in Drosophila . 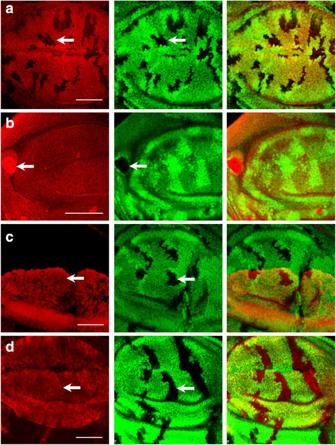Figure 1: Effects of neddylation and deneddylation on F-box proteins Slimb and Ago. (a)CSN5nullclones generated inDrosophilathird-instar larval wing discs are revealed by the absence of GFP (green). The protein level oftubulinpromoter-drivenmyc-slimb(red) decreases in GFP-negativeCSN5nullclones (arrow). (b)Nedd8AN015clones marked by the absence of GFP (green) were generated in wing discs expressing Myc-Slimb. The level of Myc-Slimb (red) inNedd8AN015clones is higher (arrow) compared with wild type. (c) The level of Myc-SlimbΔfbx (red) expressed byap-GAL4is unaltered byCSN5nullmutation (arrow) in the dorsal compartment of wing discs. (d) GFP-negativeCSN5nullclones are generated in wing discs (green), in which Flag-Ago (red) is expressed in wing pouches under the control ofms1096-GAL4.Flag-tag staining of Flag-Ago protein has a comparable signal level in wild-type andCSN5nullcells (arrow). Scale bars, 50 μm. Figure 1: Effects of neddylation and deneddylation on F-box proteins Slimb and Ago. ( a ) CSN5 null clones generated in Drosophila third-instar larval wing discs are revealed by the absence of GFP (green). The protein level of tubulin promoter-driven myc-slimb (red) decreases in GFP-negative CSN5 null clones (arrow). ( b ) Nedd8 AN015 clones marked by the absence of GFP (green) were generated in wing discs expressing Myc-Slimb. The level of Myc-Slimb (red) in Nedd8 AN015 clones is higher (arrow) compared with wild type. ( c ) The level of Myc-SlimbΔfbx (red) expressed by ap-GAL4 is unaltered by CSN5 null mutation (arrow) in the dorsal compartment of wing discs. ( d ) GFP-negative CSN5 null clones are generated in wing discs (green), in which Flag-Ago (red) is expressed in wing pouches under the control of ms1096-GAL4. Flag-tag staining of Flag-Ago protein has a comparable signal level in wild-type and CSN5 null cells (arrow). Scale bars, 50 μm. Full size image Reduction in the protein levels of Slimb and Cul1 [42] in CSN mutants could promote the accumulation of SCF Slimb substrates. This was tested by examining the protein level of a typical SCF Slimb substrate Armadillo (Arm), the Drosophila ortholog of β-catenin [13] , [27] . In line with recent reports [48] , [49] , the Arm level in CSN5 null cells is slightly but consistently higher than that in wild-type cells ( Supplementary Fig. S1 ). Deneddylation enhances Ci 155 stability We also tested how deneddylation regulates another SCF Slimb substrate Ci 155 in wing discs [13] , [27] . Unlike the increased level of Arm, the Ci 155 protein level is instead downregulated in both CSN5 null and CSN4 null mutant cells ( Fig. 2a,b ), suggesting that neddylated SCF Slimb degrades more Ci 155 , despite the reduced levels of both Cul1 [42] and the substrate receptor Slimb ( Fig. 1a ) in CSN mutants. Thus, Ci 155 proteolysis is more sensitive to the level of neddylation, but less so to the bulk concentrations of SCF Slimb components. In comparison to mutant clones in the low Hh signalling region (arrowhead in Fig. 2a ), the reduction in the Ci 155 level is more prominent in low-to-intermediate Hh signalling regions (arrow in Fig. 2a ) in which the Ci 155 protein level starts to fall but has not yet reached the basal level. Deneddylation upregulates the Ci 155 level by a post-transcriptional mechanism, as we found that the protein levels of ci-myc and HA-ci transgenes under the ms1096 - GAL4 driver are reduced in CSN mutant cells (arrow in Fig. 2c and Supplementary Fig. S2 ). Furthermore, the expression of ci-lacZ that recapitulates ci transcription remains constant in CSN5 null cells ( Fig. 2d ). 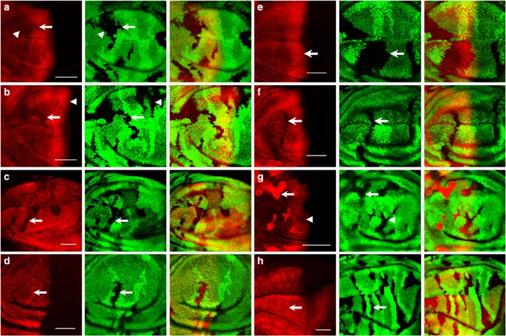Figure 2: The CSN positively regulates Ci155protein stability in wing discs. (a)CSN5nullclones are revealed by the absence of GFP (green) in wing discs. Ci155stained with the 2A1 antibody (red) is reduced inCSN5nullclones located in the A compartment, with arrow indicating mutant cells in the low-to-intermediate Hh signalling region and arrowhead indicating cells in the low Hh signalling region. (b) GFP-negativeCSN4nullclones were generated in wing discs (green). Ci155staining (red) is lower in theCSN4nullcells in the A compartment (arrow) than in the wild-type cells. The Ci155levels inCSN4nulland wild-type cells located in A/P boundary are similar (arrowhead). (c)CSN4nullclones revealed by the absence of GFP (green) were generated in wing discs that simultaneously expressUAS-ci-mycunder the control ofms1096-GAL4. Protein levels of Ci-Myc detected by the anti-Myc antibody (red) are reduced inCSN4nullmutant clones (arrow). (d) Theci-lacZexpression (red) is not reduced inCSN4nullmutant clones (arrow) generated in wing discs. (e) GFP-negativeCSN5nullclones (green) were generated in wing discs expressing wild-typeCSN5construct under the control ofms1096-GAL4. Expression of wild-type CSN5 rescues the Ci155level (red) inCSN5nullclones (arrow). (f) Expression of CSN5D148N, which loses deneddylation activity, fails to rescues the Ci155level (red) inCSN5nullclones (arrows). (g)slimbP1493,CSN5nullclones revealed by the absence of GFP (green) in wing discs show Ci155(red) accumulation in the A compartment (arrow) except when located adjacent to the A/P boundary (arrowhead). (h) The Ci-3P mutant protein (red), carrying mutations in three PKA phosphorylation sites, is ectopically expressed inCSN4nullmosaic wing pouches under the control ofms1096-GAL4.There is no difference in Ci-3P expression in wild-type and GFP-negativeCSN4nullcells (arrow). Scale bars in all panels represent 50 μm. Figure 2: The CSN positively regulates Ci 155 protein stability in wing discs. ( a ) CSN5 null clones are revealed by the absence of GFP (green) in wing discs. Ci 155 stained with the 2A1 antibody (red) is reduced in CSN5 null clones located in the A compartment, with arrow indicating mutant cells in the low-to-intermediate Hh signalling region and arrowhead indicating cells in the low Hh signalling region. ( b ) GFP-negative CSN4 null clones were generated in wing discs (green). Ci 155 staining (red) is lower in the CSN4 null cells in the A compartment (arrow) than in the wild-type cells. The Ci 155 levels in CSN4 null and wild-type cells located in A/P boundary are similar (arrowhead). ( c ) CSN4 null clones revealed by the absence of GFP (green) were generated in wing discs that simultaneously express UAS-ci-myc under the control of ms1096-GAL4 . Protein levels of Ci-Myc detected by the anti-Myc antibody (red) are reduced in CSN4 null mutant clones (arrow). ( d ) The ci-lacZ expression (red) is not reduced in CSN4 null mutant clones (arrow) generated in wing discs. ( e ) GFP-negative CSN5 null clones (green) were generated in wing discs expressing wild-type CSN5 construct under the control of ms1096-GAL4 . Expression of wild-type CSN5 rescues the Ci 155 level (red) in CSN5 null clones (arrow). ( f ) Expression of CSN5 D148N , which loses deneddylation activity, fails to rescues the Ci 155 level (red) in CSN5 null clones (arrows). ( g ) slimb P1493 , CSN5 null clones revealed by the absence of GFP (green) in wing discs show Ci 155 (red) accumulation in the A compartment (arrow) except when located adjacent to the A/P boundary (arrowhead). ( h ) The Ci-3P mutant protein (red), carrying mutations in three PKA phosphorylation sites, is ectopically expressed in CSN4 null mosaic wing pouches under the control of ms1096-GAL4. There is no difference in Ci-3P expression in wild-type and GFP-negative CSN4 null cells (arrow). Scale bars in all panels represent 50 μm. Full size image It has been shown that IκBα is less stable in CSN mutants because of the inactivation of the CSN-associated deubiquitinase USP15, rather than a deneddylation-related mechanism [50] . In the case of Ci 155 proteolysis, CSN-mediated deneddylation is indeed required for the regulation of Ci 155 levels, as expression of wild-type CSN5 , but not deneddylation-defective CSN5 D148N , restores the Ci 155 level in CSN5 null clones ( Fig. 2e,f ). Downregulation of Ci 155 in CSN mutant cells is SCF Slimb dependent, as Ci 155 accumulates in slimb P1493 CSN5 null double-mutant cells (arrow in Fig. 2g ). We noted that the Ci 155 level remains unchanged in slimb P1493 CSN5 null double-mutant clones in the anterior/posterior (A/P) boundary region (arrowhead in Fig. 2g ), in which Ci 155 is subjected to Cul3- but not SCF-mediated proteolysis [27] , [51] . The Ci 155 level in CSN4 null mutant clones that abuts the A/P boundary also remains unaltered (arrowhead in Fig. 2b ), suggesting that the CSN regulates only SCF Slimb -dependent Ci 155 proteolysis. PKA phosphorylation of Ci 155 is required for the interaction between Ci 155 and Slimb [12] , [21] , [22] , which should be important for the CSN to regulate SCF Slimb -dependent Ci 155 proteolysis. The HA-Ci-3P protein that contains three mutated PKA phosphorylation sites and resistant to SCF Slimb -mediated proteolysis [22] appears to have comparable expression levels in CSN4 null mutant and wild-type cells ( Fig. 2h ). This is in contrast to the wild-type Ci-Myc and HA-Ci that are decreased in CSN mutant cells ( Fig. 2c and Supplementary Fig. S2 ). Therefore, the CSN complex regulates the Ci 155 levels through the SCF Slimb machinery in the A compartment of wing discs, except at the A/P boundary region. CSN differentially regulates Ci 155 proteolysis To gain insights into how the CSN regulates SCF Slimb -mediated Ci 155 proteolysis, the proportions of proteolysed and stable Ci 155 along the A/P axis of wing discs were quantified. We generated random mosaic twin clones from double heterozygotes for the Cul1 EX and CSN4 null alleles, both located at chromosome 2R ( Fig. 3a ). One of the twin clones is homozygous for Cul1 EX , marked with the double-brightness of green fluorescent protein (GFP) signal, and the other twin clone is homozygous for CSN4 null , marked by the complete absence of GFP signal. Cells marked by single brightness of GFP signal are double heterozygous for Cul1 EX and CSN4 null , which are considered as wild-type control. The Ci 155 -expressing A compartment of wing pouches was divided into 12 equal regions, with the most anterior cells being in region 1 and cells receiving the highest level of Hh in region 12 ( Fig. 3b ). We measured the Ci 155 protein levels in Cul1 EX , CSN4 null and wild-type control cells in regions 1–12. The percentage of Ci 155 that has undergone SCF Slimb -dependent proteolysis in each region was calculated as the Ci 155 level in Cul1 EX cells (no proteolysis) subtracted by the Ci 155 level in double-heterozygous cells (normal proteolysis in wild-type control), which is then normalized to the Ci 155 level in Cul1 EX cells: percentage of Ci 155 proteolysis=([Ci 155 ] Cul1EX −[Ci 155 ] wild-type )/[Ci 155 ] Cul1EX . We found that the extent of SCF Slimb -dependent Ci 155 proteolysis is constantly high across regions 1–8, and gradually declines from region 8 to 12 ( Fig. 3c ). We also quantified the extents of SCF Slimb -dependent Ci 155 proteolysis in CSN4 null cells across regions 1–12 using the same methodology: percentage of Ci 155 proteolysis=([Ci 155 ] Cul1EX −[Ci 155 ] CSN4null )/[Ci 155 ] Cul1EX . Interestingly, Ci 155 proteolysis in CSN4 null cells remained similar to wild-type cells in regions 1–8, and graded Ci 155 proteolysis in CSN4 null cells was also present from regions 8 to 12. Remarkably, Ci 155 proteolysis is prominently enhanced in CSN4 null cells in regions 9, 10 and 11 compared with wild-type cells in the same regions, with 30, 40 and 24% reductions in the Ci 155 levels, respectively ( Fig. 3c ). In region 12 closest to the A/P boundary in which the protein level of Ci 155 is regulated by the Cul3-organized CRL [27] , [51] , the proportion of SCF Slimb -dependent Ci 155 proteolysis is unaltered in CSN4 null mutant cells (arrow in Fig. 3a and arrowhead in Fig. 2b ). Mild enhancements of 1–6% of Ci 155 proteolysis were noted in CSN4 null cells in regions 1–8, although these differences were not statistically significant except for regions 6 and 7 ( n ≥6, P <0.05 by Student's t -test). On the basis of the proteolytic curves of Ci 155 in wild-type and CSN4 null cells, we propose that proteolysis-resistant Ci 155 in wild-type cells is composed of 'stable' and 'conditionally stable' forms, the latter being stable in wild-type cells but proteolysed in CSN mutant cells by SCF Slimb , whereas the former is insensitive to the absence of CSN activity. The levels of conditionally stable Ci 155 are highest in regions 9–11, in which cells are exposed to low-to-intermediate levels of Hh. 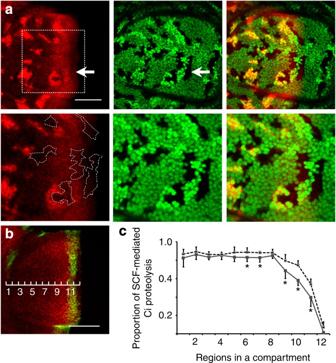Figure 3: The CSN regulates Ci155proteolysis predominantly in intermediate Hh signalling regions. (a) Mutant clones forCSN4nullorCul1EXwere generated simultaneously in the same wing discs of thehsflp;FRT42D CSN4null/FRT42D Cul1EX,nlsGFPgenotype. Ci155(red) levels stained by 2A1 antibody was measured in the following cells:CSN4nullmutant clones marked by the absence of GFP,Cul1EXmutant clones marked by two copies of GFP and double-heterozygousCSN4null/+,Cul1EX/+cells marked by one copy of GFP (green). The lower panels inashow close-up images of a region near the A/P boundary (outlined by a dashed square in upper left panel), with someCSN4nullclones highlighted by white dashed lines (lower left panel). (b) The A compartment of wing pouches showing expression of Ci155(red) anddpp-lacZ(green) is divided equally into 12 regions along the A/P axis. Expression ofdpp-lacZis detected in region 11. Scale bars represent 50 μm (a,b). (c) The portions of Ci155that undergo SCFSlimb-mediated proteolysis in regions 1–12 of wild-type (grey line) andCSN4nullmutant cells (dashed line) were calculated. Averaged Ci155pixel intensities for each region (n>= 6) are shown. Asterisks indicate a significant difference of Ci155proteolysis between wild-type andCSN4null(P<0.05). Error bars present the standard deviation. Figure 3: The CSN regulates Ci 155 proteolysis predominantly in intermediate Hh signalling regions. ( a ) Mutant clones for CSN4 null or Cul1 EX were generated simultaneously in the same wing discs of the hsflp ; FRT42D CSN4 null / FRT42D Cul1 EX , nlsGFP genotype. Ci 155 (red) levels stained by 2A1 antibody was measured in the following cells: CSN4 null mutant clones marked by the absence of GFP, Cul1 EX mutant clones marked by two copies of GFP and double-heterozygous CSN4 null/+ , Cul1 EX/+ cells marked by one copy of GFP (green). The lower panels in a show close-up images of a region near the A/P boundary (outlined by a dashed square in upper left panel), with some CSN4 null clones highlighted by white dashed lines (lower left panel). ( b ) The A compartment of wing pouches showing expression of Ci 155 (red) and dpp-lacZ (green) is divided equally into 12 regions along the A/P axis. Expression of dpp-lacZ is detected in region 11. Scale bars represent 50 μm ( a , b ). ( c ) The portions of Ci 155 that undergo SCF Slimb -mediated proteolysis in regions 1–12 of wild-type (grey line) and CSN4 null mutant cells (dashed line) were calculated. Averaged Ci 155 pixel intensities for each region ( n >= 6) are shown. Asterisks indicate a significant difference of Ci 155 proteolysis between wild-type and CSN4 null ( P <0.05). Error bars present the standard deviation. Full size image CSN is required for Hh-dependent wing patterning To examine whether the level of conditionally stable Ci 155 is essential for distinct cell fates directed by graded Hh signalling, we assayed the activation of Hh-responsive, position-specific genes, such as ptc and dpp , whose expression represent high and low Hh signalling responses, respectively [19] . Interestingly, we found that the expression of dpp-lacZ is significantly repressed in CSN4 null mutant cells (arrow in Fig. 4a ), whereas the Ptc protein level and the expression of ptc-lacZ remain unaltered (arrows in Fig. 4b,c ), indicating a critical role of the conditionally stable Ci 155 for the Hh-mediated dpp expression. The expression of e ngrailed ( en ) is regulated by high Hh signalling activity in the A/P boundary [52] . We tested whether en expression in the A/P boundary is downregulated in CSN4 null mutant because of Ci 155 proteolysis. En protein level is instead enhanced not only at the A/P boundary but also in A and P compartments, in which en expression is independent from Hh signalling ( Fig. 4d ), suggesting that en expression is subjected to another layer of regulation by the CSN. 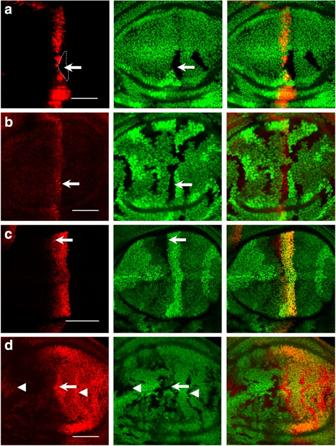Figure 4: The CSN differentially regulates Hh downstream gene expression. (a) ACSN4nullclone (indicated by the dashed outline) is generated indpp-lacZwing discs.dpp-lacZexpression detected by anti-β-gal antibody (red) is markedly repressed inCSN4nullcells (arrow). (b)CSN5nullclones indicated by the absence of GFP are generated in wing discs. Ptc (red) protein level inCSN5nullcells (arrow) detected by the monoclonal antibody Apa-1 is similar to that in wild-type cells. (c)ptc-lacZstaining (red) is comparable in wild-type andCSN5nullcells that are marked by the absence of GFP (arrow). (d) En protein levels (red) are increased in theCSN5nullcells (arrow) located in the A/P boundary as well as in the A and P compartments (arrowheads). Scale bars in all panels represent 50 μm. Figure 4: The CSN differentially regulates Hh downstream gene expression. ( a ) A CSN4 null clone (indicated by the dashed outline) is generated in dpp-lacZ wing discs. dpp-lacZ expression detected by anti-β-gal antibody (red) is markedly repressed in CSN4 null cells (arrow). ( b ) CSN5 null clones indicated by the absence of GFP are generated in wing discs. Ptc (red) protein level in CSN5 null cells (arrow) detected by the monoclonal antibody Apa-1 is similar to that in wild-type cells. ( c ) ptc-lacZ staining (red) is comparable in wild-type and CSN5 null cells that are marked by the absence of GFP (arrow). ( d ) En protein levels (red) are increased in the CSN5 null cells (arrow) located in the A/P boundary as well as in the A and P compartments (arrowheads). Scale bars in all panels represent 50 μm. Full size image To further substantiate the notion that small perturbations of the Ci 155 level can inactivate dpp expression, we tested whether ms1096-GAL4 -driven ci-RNAi [53] could abolish dpp-lacZ expression. The ms1096-GAL4 driver exhibits differential expression in wing pouches, with higher levels in the dorsal and lower levels in the ventral compartment. As a consequence, dpp-lacZ expression is detectable in the ventral compartment, but diminished in the dorsal compartment, in which the Ci 155 level is comparably reduced as in CSN5 null cells ( Supplementary Fig. S3 ). In contrast, the expression of ptc-lacZ remains unaltered in the dorsal compartment ( Supplementary Fig. S3 ). Therefore, the dpp-lacZ expression is sensitive to small reductions in Ci 155 levels. The expression of dpp-lacZ is downregulated by Ci 75 , the transcriptional repressor produced by SCF Slimb -mediated proteolysis of Ci 155 , whereas Ptc expression is not [54] . Disruption of dpp-lacZ but not Ptc expression in CSN mutant cells suggests an alternative possibility that a higher level of Ci 75 accumulates in CSN mutant cells as a result of SCF Slimb -mediated proteolysis. Proper phosphorylation confers conditionally stable Ci 155 Our results suggest that low-to-intermediate Hh signalling (regions 9–11) renders the appearance of conditionally stable Ci 155 , whereas high (region 12) and low (regions 1–8) Hh signalling activities do not. It has also been suggested that graded Hh signalling activities counteract Ci 155 proteolysis by inhibiting different levels of Ci 155 phosphorylation [55] , leading to differential affinities to the F-box protein Slimb for SCF Slimb -mediated proteolysis [26] . We therefore tested whether the phosphorylation status of Ci 155 alters the level of conditionally stable Ci 155 . Ci 155 phosphorylation can be compromised by the ectopic expression of dominant-negative GSK3β (DN-GSK3β), resulting in the inhibition of Ci 155 proteolysis in the low Hh signalling region [24] . Although proteolysed Ci 155 in the low Hh region (regions 1–8) is 84±5% of total Ci 155 in wild-type cells ( Fig. 3c ), it is reduced to 38±8% in the DN-GSK3β expression clones (averaged from seven clones in regions 1–8, arrowhead in Fig. 5a ). Accumulation of Ci 155 in regions 1–8, however, is suppressed by the CSN4 null mutation (arrow in Fig. 5a ), with 75±11% of Ci 155 undergoing proteolysis in CSN4 null mutant cells expressing DN-GSK3β ( n =8). Thus, the accumulated Ci 155 in regions 1–8 on DN - GSK3β β wings is conditionally stable in nature, undergoing proteolysis in the absence of CSN activity. Likewise, inhibiting CKI kinase activity by expressing dominant-negative Doubletime (DN-DBT) causes Ci 155 accumulation [25] , which is also suppressed by the CSN4 null mutation, as shown by reduced Ci 155 levels in CSN4 null mutant cells expressing DN-DBT (arrow, Fig. 5b ) compared with wild-type cells expressing DN-DBT . Thus, lowering the phosphorylation level by inhibiting either GSK3β or CKI produces conditionally stable Ci 155 in the low Hh signalling region, mimicking the Ci 155 behaviour in the region with low-to-intermediate Hh signalling. 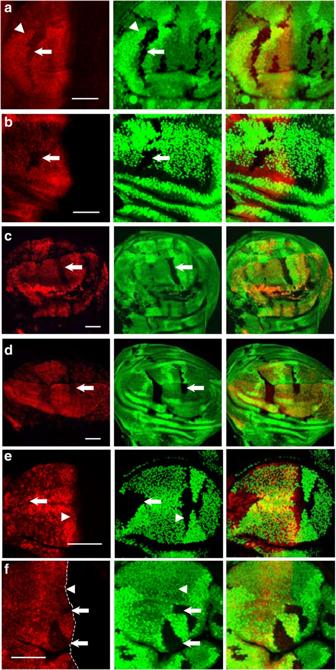Figure 5: Conditionally stable Ci155is sensitive to phosphorylation levels. (a)CSN4nullclones are generated in wing discs that express dominant-negative GSK3β (DN-GSK3β) byms-1096-GAL4. DN-GSK3β increases Ci155expression (red) in low Hh signalling regions (arrowhead). The Ci155level is downregulated inCSN4nullcells (arrow) in the presence of DN-GSK3β. (b) Inhibition of CKI activity byC765-GAL4-driven DN-DBT increases the accumulation of Ci155(red) in wild-type cells. This accumulation of Ci155is downregulated inCSN4nullclones (arrow). (c)CSN4nullclones marked by the absence of GFP (green) were generated in wing discs expressingUAS-ci-C1-3E-mycunder the control ofms1096-GAL4. The Ci-C1-3E-Myc levels detected by anti-Myc antibody (red) were decreased inCSN4nullclones (arrow). (d)CSN4nullclones marked by the absence of GFP (green) were generated in wing discs expressingUAS-ci-G2-3E-myc. Ci-G2-3E-Myc (red) staining is decreased inCSN4nullclones (arrow). (e) Ectopic expression of PKA-R*, the regulatory subunit of PKA, byC765-GAL4increases Ci155levels in the A compartment. The upregulated Ci155levels (red) either in low or low-to-intermediate Hh regions (arrow and arrowhead, respectively) are not altered inCSN5nullclones in wing discs. (f)CSN5nullclones were generated in wing discs that express the catalytic subunit of PKA (PKA-mC*) byms-1096-GAL4. Ci155levels (red) near the A/P boundary in the high Hh signalling region is downregulated inCSN5nullclones (arrows) compared with wild-type cells (arrowhead). Dashed lines indicate the A/P boundary. Scale bars in all panels represent 50 μm. Figure 5: Conditionally stable Ci 155 is sensitive to phosphorylation levels. ( a ) CSN4 null clones are generated in wing discs that express dominant-negative GSK3β (DN-GSK3β) by ms-1096-GAL4 . DN-GSK3β increases Ci 155 expression (red) in low Hh signalling regions (arrowhead). The Ci 155 level is downregulated in CSN4 null cells (arrow) in the presence of DN-GSK3β. ( b ) Inhibition of CKI activity by C765-GAL4 -driven DN-DBT increases the accumulation of Ci 155 (red) in wild-type cells. This accumulation of Ci 155 is downregulated in CSN4 null clones (arrow). ( c ) CSN4 null clones marked by the absence of GFP (green) were generated in wing discs expressing UAS-ci-C1-3E-myc under the control of ms1096-GAL4 . The Ci-C1-3E-Myc levels detected by anti-Myc antibody (red) were decreased in CSN4 null clones (arrow). ( d ) CSN4 null clones marked by the absence of GFP (green) were generated in wing discs expressing UAS-ci-G2-3E-myc . Ci-G2-3E-Myc (red) staining is decreased in CSN4 null clones (arrow). ( e ) Ectopic expression of PKA-R*, the regulatory subunit of PKA, by C765-GAL4 increases Ci 155 levels in the A compartment. The upregulated Ci 155 levels (red) either in low or low-to-intermediate Hh regions (arrow and arrowhead, respectively) are not altered in CSN5 null clones in wing discs. ( f ) CSN5 null clones were generated in wing discs that express the catalytic subunit of PKA (PKA-mC*) by ms-1096-GAL4 . Ci 155 levels (red) near the A/P boundary in the high Hh signalling region is downregulated in CSN5 null clones (arrows) compared with wild-type cells (arrowhead). Dashed lines indicate the A/P boundary. Scale bars in all panels represent 50 μm. Full size image To examine the critical role of phosphorylation in the appearance of conditionally stable Ci 155 , we examined whether the CSN regulates the protein levels of Ci mutants in which CKI or GSK3β phosphorylation sites are mutated (Ci-C1-3E and Ci-G2-3E, respectively). Both Ci-C1-3E and Ci-G2-3E cannot be proteolysed efficiently in the absence of Hh signalling [26] . When ectopically expressed in wing pouches by ms1096-GAL4 , the protein levels of Ci-C1-3E or Ci-G2-3E are downregulated by the CSN4 null mutation (arrows in Fig. 5c,d ), suggesting that Ci-C1-3E and Ci-G2-3E represent the CSN-regulated, conditionally stable forms of Ci. Expression of the PKA regulatory subunit, PKA-R*, inhibits PKA-dependent Ci 155 phosphorylation and precludes PKA-primed sites for further GSK3β and CKI phosphorylation [21] . We therefore examined the effect of further reducing Ci 155 phosphorylation on the CSN-dependent Ci 155 stabilization. Under the control of C765-GAL4 , the PKA-R* expression enhances Ci 155 levels across the A compartment. However, no downregulation of Ci 155 levels could be detected in CSN4 null mutant cells expressing PKA-R* , including those in intermediate-to-high and low Hh signalling regions (arrowhead and arrow in Fig. 5e , respectively). Therefore, phosphorylation-depleted Ci 155 is unlikely to be the CSN-regulated conditionally stable form. The above analysis also suggests that lack of PKA phosphorylation in the high Hh signalling region 12 may account for the absence of conditionally stable Ci 155 . To test this, Ci 155 phosphorylation by PKA is induced by expressing the catalytic subunit mC* under the control of ms1096-GAL4 [23] . Expression of mC* equalizes Ci 155 levels across the A compartment, mainly because of the downregulation of Ci 155 levels in intermediate-to-high Hh signalling regions and the upregulation in high Hh signalling region 12. However, the Ci 155 levels in mC*-expressing CSN5 null mutant clones were reduced in large clones covering region 12 (arrows in Fig. 5f ), as compared with mC*-expressing wild-type cells (arrowhead in Fig. 5f ), an indication of the appearance of conditionally stable Ci 155 even in the presence of high Hh signalling. Given that conditionally stable Ci 155 appears in the low Hh signalling region on GSK3β or CKI inhibition and in the high Hh signalling region by PKA activation, these results support the idea that partially phosphorylated Ci 155 represents the conditionally stable form regulated by the CSN. Dominant-negative SlimbΔfbx fails to induce CSN regulation To further corroborate the SCF-dependent mechanism for CSN regulation, we tested whether Ci 155 has to be incorporated into the SCF complex for the CSN to confer its conditional stability. To do this, the F-box-truncated SlimbΔfbx protein that can competitively bind Ci 155 but cannot be incorporated into SCF was ectopically expressed by ap-GAL4 in wing discs. Higher levels of Ci 155 detected in wing discs suggest that SlimbΔfbx-sequestered Ci 155 is free from SCF-mediated proteolysis. Unlike the conditionally stable Ci 155 upregulated by DN-GSK3β or DN-DBT expression, the upregulated Ci 155 levels caused by SlimbΔfbx expression is insensitive to the absence of CSN activity in CSN5 null cells (arrow, Fig. 6a ). Thus, Ci 155 that binds the substrate receptor Slimb, but fails to form SCF Slimb -Ci 155 intermediates, is insufficient to produce conditionally stable Ci 155 . 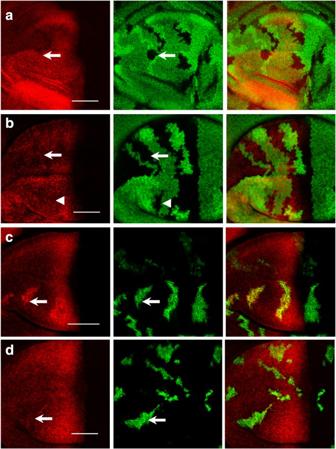Figure 6: CSN control of Ci155levels upregulated by SlimbΔfbx or Uba1 depletion. (a)CSN5nullclones are generated in wing discs expressing Myc-SlimbΔfbx in the dorsal compartment under the control ofap-GAL4. Ectopic expression of SlimbΔfbx increases the levels of Ci155(red) in the dorsal compartment. Moreover, the upregulated Ci155is maintained inCSN5nullclones (arrow). (b) Under the control ofms1096-GAL4,the moderate level of ectopic Myc-SlimbΔfbx in the dorsal compartment causes similar accumulation of Ci155(red) in both wild-type andCSN5nullcells (arrowhead); the lower level of ectopic Myc-SlimbΔfbx in the ventral compartment also causes similar accumulation of Ci155in both wild-type andCSN5nullcells (arrow) (c) GFP-marked MARCM clones (green) expressinguba1-dsRNAbyms1096-GAL4generated in wing discs show upregulation of Ci155(red) levels compared with adjacent wild-type cells that are negative for GFP. (d) GFP-markeduba1-dsRNAMARCM clones that are alsoCSN5nullshow Ci155levels (red) comparable with adjacent GFP-negative wild-type cells. Scale bars in all panels represent 50 μm. Figure 6: CSN control of Ci 155 levels upregulated by SlimbΔfbx or Uba1 depletion. ( a ) CSN5 null clones are generated in wing discs expressing Myc-SlimbΔfbx in the dorsal compartment under the control of ap-GAL4 . Ectopic expression of SlimbΔfbx increases the levels of Ci 155 (red) in the dorsal compartment. Moreover, the upregulated Ci 155 is maintained in CSN5 null clones (arrow). ( b ) Under the control of ms1096-GAL4, the moderate level of ectopic Myc-SlimbΔfbx in the dorsal compartment causes similar accumulation of Ci 155 (red) in both wild-type and CSN5 null cells (arrowhead); the lower level of ectopic Myc-SlimbΔfbx in the ventral compartment also causes similar accumulation of Ci 155 in both wild-type and CSN5 null cells (arrow) ( c ) GFP-marked MARCM clones (green) expressing uba1 - dsRNA by ms1096-GAL4 generated in wing discs show upregulation of Ci 155 (red) levels compared with adjacent wild-type cells that are negative for GFP. ( d ) GFP-marked uba1 - dsRNA MARCM clones that are also CSN5 null show Ci 155 levels (red) comparable with adjacent GFP-negative wild-type cells. Scale bars in all panels represent 50 μm. Full size image Although SlimbΔfbx-sequestered Ci 155 is insensitive to the CSN regulation, the residual Ci 155 protein that is free from SlimbΔfbx titration is still insensitive to the CSN regulation, arguing that the CSN regulation does not increase the concentration or availability of the SCF Slimb -Ci 155 intermediate. As the strong expression of SlimbΔfbx by ap-GAL4 might sequester Ci 155 from SCF regulation, ms1096-GAL4 was used to express moderate levels of SlimbΔfbx in the dorsal compartment and low levels in the ventral compartment. Moderate depletion of the SCF Slimb -Ci 155 intermediates in the dorsal compartment by ms1096-GAL4 behaved similarly to the strong depletion by ap-GAL4 ; no significant difference in Ci 155 proteolysis was detected between wild-type and CSN5 null cells (arrowhead in Fig. 6b ). Interestingly, although the Ci 155 levels fluctuate in the ventral compartment because of weak depletion of the SCF Slimb -Ci 155 intermediates, they were still insensitive to any CSN modulation (arrow in Fig. 6b ). In these experiments, the remaining Ci 155 after SlimbΔfbx titration still possessed a high affinity for Slimb in low Hh signalling regions. Thus, in contrast to the perturbation by DN-GSK3β, different extents of perturbation on the concentration of tightly associated SCF Slimb -Ci 155 intermediates are invariantly insufficient to generate conditionally stable Ci 155 . Sensitivity of Ci 155 proteolysis to the Ub supply A compromised affinity between partially phosphorylated Ci 155 and Slimb can result in reduced availability of SCF Slimb -Ci 155 intermediates. However, as shown in the SlimbΔfbx titration experiment, reduced availability of SCF Slimb -Ci 155 intermediates was insufficient to confer CSN regulation. We hypothesized that partial Ci 155 phosphorylation may compromise the duration of SCF Slimb -Ci 155 association, disrupting substrate polyubiquitylation. In line with this idea, recent findings suggest that most of the encounters between SCF and its substrate are unproductive, with the dissociation rate k off being much larger than the reaction rate of adding the first Ub ( k ub1 ) [38] . Although most of the encounters between SCF and its substrate are unproductive, neddylation of SCF allows polyubiquitylation ( k ub2–4 ) to proceed at higher rates once the first Ub is added [38] . Therefore, CSN deneddylation could be critical at the Ub chain elongation step when the affinity between SCF and substrate is reduced, such as in the case of partially phosphorylated Ci 155 . Processive Ci 155 ubiquitylation would demand a constant supply of activated Ub, which could be sensitive to the level of the Ub-activating enzyme. In mosaic analysis with a repressible cell marker (MARCM) clones, in which uba1-dsRNA was expressed to knockdown the expression of the Ub-activating enzyme, accumulation of Ci 155 (arrow in Fig. 6c ) suggests that the insufficiency in supplying activated Ub leads to the disruption of Ci 155 polyubiquitylation and proteolysis. The defect of Ci 155 accumulation in uba1-dsRNA cells is likely caused by reduced ubiquitylation, which could be compensated by constitutively neddylated SCF that promotes processivity of ubiquitylation. Indeed, the elevated Ci 155 level in uba1 - dsRNA knockdown cells was almost completely suppressed by introducing the CSN5 null mutation in the uba1 - dsRNA MARCM clones (arrow in Fig. 6d ). This result is consistent with the idea that inactivating the deneddylation machinery could compensate for inefficient polyubiquitylation in uba1 - dsRNA knockdown cells, thereby restoring the assembly of proteasome-targeting polyubiquitin chains on Ci 155 . In this study, we show that CSN-mediated deneddylation of SCF Slimb is critical for the Ci 155 stability in low-to-intermediate Hh regions in which partially phosphorylated Ci 155 has a reduced affinity for the ubiquitylation machinery SCF Slimb . The effect of CSN deneddylation on SCF Slimb likely reduces ubiquitylation processivity, thus preserving 'conditionally stable Ci 155 ' in these low-to-intermediate Hh regions. We propose a broader view for CRL substrate degradation in vivo , determined by three interdependent factors: substrate-enzyme affinity, deneddylation-regulated CRL activity and the supply of Uba1-activated Ub. We propose that steady-state Ci 155 levels are low in the low Hh signalling regions because processive polyubiquitylation of the tightly associated SCF Slimb -Ci 155 complex proceeds even with intermittent SCF Slimb inactivation by CSN-mediated deneddylation ( Fig. 7a ). In low-to-intermediate Hh regions, the steady-state Ci 155 levels are sensitive to CSN-mediated deneddylation as a result of weakened SCF Slimb -Ci 155 association, as in DN-GSK3β cells ( Fig. 7b ). In uba1-dsRNA cells, the Ci 155 levels are sensitive to CSN-mediated deneddylation because of insufficient activated Ub ( Fig. 7c ). In these cases, we envision that processive polyubiquitylation becomes more difficult because of constant neddylation–deneddylation cycling by the CSN, and can be aborted by the dissociation of Ci 155 from weakly associated SCF Slimb -Ci 155 or the lack of activated Ub. However, an insufficiency in Ci 155 downregulation can be offset by constitutive neddylated SCF Slimb in CSN mutants, which ubiquitylates substrates processively on a single SCF Slimb -Ci 155 encounter ( Fig. 7d,e ). This model explains the expression of CSN-dependent conditionally stable Ci 155 in the low-to-intermediate Hh signalling regions, in which Ci 155 may be released from the labile SCF Slimb -Ci 155 complex before SCF re-neddylation. 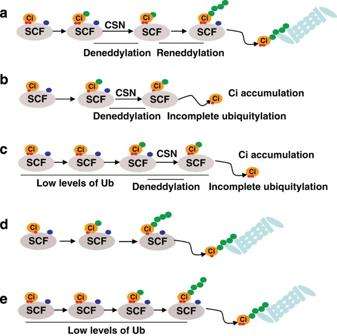Figure 7: Models for SCFSlimb-mediated Ci155proteolysis. Successful substrate polyubiquitylation requires collaboration of three components: adequate substrate–enzyme interaction time, persistent neddylated E3 ligase activity and high levels of activated ubiquitin supply. Green dot, ubiquitin; blue dot, Nedd8; and red dot, phosphate group. (a) For fully phosphorylated Ci155that binds strongly to SCF in no-to-low Hh signalling regions, long substrate–enzyme binding duration allows complete polyubiquitylation, despite temporary inactivation of SCF ligase by CSN-mediated deneddylation. (b) In low-to-intermediate Hh signalling regions as well as in the presence of DN-GSK3β, partially phosphorylated Ci155associates with SCF weakly. Dissociation of Ci155from the SCFSlimbcomplex following CSN-mediated deneddylation of SCF disrupts processive ubiquitylation of Ci155. (c) Limited supply of activated ubiquitin could disrupt processive ubiquitylation of fully phosphorylated Ci155in no-to-low Hh regions in the presence of CSN deneddylation. (d)CSNmutations allow the processivity of polyubiquitylation mediated by constantly neddylated SCF, which compensates for the short duration of interaction between SCFSlimband Ci155in low-to-intermediate Hh signalling regions or in the presence of DN-GSK3β. (e) In no-to-low Hh regions, limited supply of activated ubiquitin inuba1-dsRNAcells interrupts Ci155polyubiquitylation, which is suppressed by constitutively neddylated SCF inCSNmutants. Figure 7: Models for SCF Slimb -mediated Ci 155 proteolysis. Successful substrate polyubiquitylation requires collaboration of three components: adequate substrate–enzyme interaction time, persistent neddylated E3 ligase activity and high levels of activated ubiquitin supply. Green dot, ubiquitin; blue dot, Nedd8; and red dot, phosphate group. ( a ) For fully phosphorylated Ci 155 that binds strongly to SCF in no-to-low Hh signalling regions, long substrate–enzyme binding duration allows complete polyubiquitylation, despite temporary inactivation of SCF ligase by CSN-mediated deneddylation. ( b ) In low-to-intermediate Hh signalling regions as well as in the presence of DN-GSK3β, partially phosphorylated Ci 155 associates with SCF weakly. Dissociation of Ci 155 from the SCF Slimb complex following CSN-mediated deneddylation of SCF disrupts processive ubiquitylation of Ci 155 . ( c ) Limited supply of activated ubiquitin could disrupt processive ubiquitylation of fully phosphorylated Ci 155 in no-to-low Hh regions in the presence of CSN deneddylation. ( d ) CSN mutations allow the processivity of polyubiquitylation mediated by constantly neddylated SCF, which compensates for the short duration of interaction between SCF Slimb and Ci 155 in low-to-intermediate Hh signalling regions or in the presence of DN-GSK3β. ( e ) In no-to-low Hh regions, limited supply of activated ubiquitin in uba1-dsRNA cells interrupts Ci 155 polyubiquitylation, which is suppressed by constitutively neddylated SCF in CSN mutants. Full size image Substrate–SCF affinity is controlled by substrate phosphorylation and, in the case of Ci 155 , the number of phospho groups on substrates. It was predicted that switch-like protein degradation could be achieved for substrates bearing multiple phosphorylation sites. For example, SCF-mediated Sic1 polyubiquitylation and degradation ensues at the G1–S transition when the number of phosphorylated sites on Sic1 reaches six, as Sic1 binding affinity to the F-box protein CDC4 increases dramatically from Sic1-5p to Sic1-6p [56] . Ci 155 also bears multiple phosphorylation sites. Unlike Sic1, however, partial phosphorylation of Ci 155 is meaningful in establishing low-to-intermediate responses to Hh signalling. The amount of Ci 155 binding to Slimb increases incrementally with the number of phosphorylated sites [26] , which precludes decisive proteolysis and allows the meta-stable SCF Slimb -Ci 155 intermediates for CSN regulation. In CSN mutant wing discs, responses to Hh signalling become more switch-like, as only low and high Hh signalling responses are detected. Thus, this study and previous studies [23] , [24] , [25] , [26] , [57] indicate that partial phosphorylation of Ci 155 is essential, but not sufficient, for non-switch-like substrate proteolysis. CSN-mediated deneddylation has to be incorporated into the machinery for specific enhancement of Ci 155 levels over a low threshold. Whether it is the enhanced levels of Ci 155 or the reduced levels of the proteolysed Ci 75 repressor that affect dpp-lacZ expression is unclear. This specific requirement of deneddylation in developing wings underscores the developmental role of CSN deneddylation at a tissue level. We also envision that CSN-mediated deneddylation of cullin-based ligases may modulate cellular levels of many other proteins in a context-dependent manner, thereby adjusting their biological readouts to meet distinct requirements of different cell contexts in a multicellular organism. Fly genetics and fly stocks Cul1 EX [12] , Nedd8 AN015 [12] , UAS-CSN5 [42] , UAS-CSN5 D148N [42] and UAS-flag-ago [58] ; CSN4 null and CSN5 null [59] ; UAS-HA-ci-3P [22] , Tub-myc-slimb , UAS-myc-slimb- Δ fbx [47] , UAS-DN-GSK3β [24] , UAS-DN-DBT [25] , UAS-ci-myc [26] , UAS-ci-C1-3E-myc [26] , UAS-ci-G2-3E-myc [26] and slimb P1493 [13] ; UAS-PKA-R* and UAS-PKA-mC* [60] have been described previously. BS3.0 dpp-LacZ and ci-LacZ were obtained from Bloomington stock center. UAS-uba1-dsRNA (stock ID: 1782R-2) was obtained from Fly Stocks of National Institute of Genetics. hsflp ; FRT42D ubi-nlsGFP ; C765-GAL4/TM6B , ms1096-GAL4 , hsflp ; FRT42D ubi-nlsGFP , hsflp ; ap-GAL4/CyO ; FRT82B ubi-nlsGFP and ms1096-GAL4 , hsflp ; FRT82B ubi-nlsGFP were used to generate CSN4 null and CSN5 null mutant clones that simultaneously express transgenes of interest. ms1096-GAL4 , hsflp ; FRT82B tub-GAL80 was used to generate CSN5 null MARCM clones in wing pouches. hsflp/+ , FRT42D Cul1 EX , ubi-nlsGFP/FRT42D CSN4 null was used to generate twin mutant clones for Cul1 EX and CSN4 null . ms1096-GAL4 , hsflp/+ ; FRT42D Cul1 EX , ubi-nlsGFP/FRT42D CSN4 null ; UAS-DN-GSK3β/+ was used to generate twin mutant clones for Cul1 EX and CSN4 null in DN-GSK3β -expressing wing discs. Flies were kept at 25 °C. At 48–72 h after egg laying, larvae were heat shocked at 37 °C for 1 h to generate CSN4 null and CSN5 null mutant clones. To generate uba1-shRNA -expressing CSN5 null MARCM clones, 72 h after egg laying, ms1096-GAL4 , hsflp/+ ; UAS-uba1-dsRNA/+ ; FRT82B CSN5 null /FRT82B tub-GAL80 larvae were heat shocked at 37 °C for 1 h. Immunostaining and image processing For immunostaining, dissected imaginal wing discs from wandering third-instar larvae were fixed in 4% formaldehyde in phosphate-buffered saline (PBS) solution for 17 min, washed with 0.3% triton X-100 in PBS (PBST) for 10 min (three times), blocked in PBST supplemented by 5% normal donkey serum for 30 min and incubated with primary antibodies of various dilutions in PBST containing 5% normal donkey serum for 16 h at 4 °C. These imaginal discs were washed with PBST for 10 min (three times), followed by a 2-h secondary antibody incubation before washes (three times in PBST). The stained wing discs were mounted on slides in PBS + 50% glycerol. All procedures were performed at 25 °C unless specifically described. The primary antibodies used were mouse anti-Flag (M2, 1:3,000; Sigma), mouse anti-Myc (9E10, 1:200; Santa Cruz Biotechnology), rat anti-full-length Ci (2A1, 1:10; Developmental Studies Hybridoma Bank), mouse anti-β-gal (1:1,000; Sigma) and mouse anti-Arm and mouse anti-En (1:100, N2-7A1 and 1:30, 4D9, respectively, Developmental Studies Hybridoma Bank). The secondary antibodies used were Cy3-conjugated goat anti-mouse IgG, Cy3-conjugated goat anti-rabbit IgG and Cy3-conjugated goat anti-rat IgG (1:1,000, Jackson ImmunoResearch Laboratories). Images were acquired by Zeiss LSM510 META Confocal Imaging System (Zeiss). To quantify Ci 155 expression levels in wild-type, CSN4 null and Cul1 EX cells, the maximal pixel intensities of Ci 155 immunoreactivities in the A compartment were below 255 and set to be zero in the P compartment as background control by using Photoshop (Adobe). How to cite this article: Wu, J.-T. et al . CSN-mediated deneddylation differentially modulates Ci 155 proteolysis to promote Hedgehog signalling responses. Nat. Commun. 2:182 doi: 10.1038/ncomms1185 (2011).